Spin regulation in composite spin-filter barrier devices Magnetic insulators are known to provide large effective Zeeman fields that are confined at an interface, making them especially powerful in modifying adjacent one- or two-dimensional electronic structures. Utilizing this phenomenon and the other important property of magnetic insulators—spin filtering—here we report the generation and subsequent detection of a large interface field, as large as tens of tesla in EuS/Al/EuS heterostructures with metallic coulomb islands confined within a magnetic insulator barrier. The unique energy profile across this sandwich structure produces spin-assisted charge transfer across the device, generating a spontaneous spin current and voltage. These unique properties can be practical for controlling spin flows in electronic devices and for energy harvesting. Incorporating electron spin degree of freedom makes it possible to create novel functionality and flexibility in electronic devices. This is known as spintronics, where the goal is to meet the ever demanding needs of information technology. One of the core challenges lies in lifting the spin degeneracy in an otherwise non-magnetic system, and the subsequent extraction of spin-resolved signals. Tremendous progress has been made towards these goals, for examples, the discovery of normal and inversed spin Hall effect [1] , [2] , [3] , [4] where the travelling spins are naturally distinguished by spin–orbit interactions; the direct injection and transport of spin carriers in metallic and semiconducting media [5] , [6] , [7] where one can further manipulate the spins through field effects [8] , [9] , [10] . To address the challenge of generation and detection of spin signals, we focus our attention to a special class of materials—magnetic insulators, which are best known for their ability to selectively allow the passage of only one type of spin through them, namely the spin-filtering (SF) effect [11] . Therefore they can be readily used for directly probing spin information in transport studies. SF is a generic property exhibited by any magnetic insulator, whose conduction band is spin split by an exchange interaction. Owing to the exponential dependence of the quantum-tunnelling probability on tunnel barrier heights, a tunnel barrier formed with a magnetic insulator is highly efficient in selecting transient electrons according to their spin types, hence the name SF. When an electron attempts to tunnel across a SF barrier, its tunnelling probability is strongly dependent on its relative spin orientation with respect to the magnetic orientation of the SF barrier. Generally speaking, the electrons with their spin aligned parallel to the SF barrier see a lower tunnel barrier height and thus tunnel through more readily than electrons with the opposite spin. Utilization of magnetic insulators in the SF process, observed four decades ago [12] , [13] , is receiving renewed attention today [11] , [14] . By employing the SF phenomenon, large spin polarization has been directly generated from non-magnetic electrodes [15] , [16] , and sizeable magnetoresistance (MR) has been realized in quasi-SF tunnel junctions that utilize one ferromagnetic electrode [17] , [18] , as well as in double SF tunnel junctions consisting of non-magnetic electrodes [19] . Recent room temperature operation of the SF effect [20] has generated further excitement in the field for their device application potential. Furthermore, conduction electrons travelling near the interface of a magnetic insulator experience indirect exchange interactions [21] with the localized-magnetic moments at the interface and become spin split in the process. Very strong exchange interaction does occur at the interface between rare-earth compounds and metals [22] , [23] , [24] , [25] , [26] . The highly localized and ferromagnetically ordered 4 f electrons in the rare-earth ions can induce magnetic orientation of conduction electrons at the interface of neighbouring metals, giving rise to large spin splitting within the metal conduction bands. This leads to an effective interfacial exchange field between a magnetic insulator and its proximate electron gas, and is considered an efficient way to generate extremely large ‘effective’ Zeeman fields that is particularly efficient in low-dimensional electronic structures. Europium sulphide (EuS), a rare-earth chalcogenide, conveniently exhibits both phenomena. Here we report a method to harvest spin information by combining the dual functionalities of magnetic insulators in a single EuS/Al/EuS transport device. The unique spin-dependent energy profiles across the double magnetic insulator barriers regulate any non-equilibrium perturbation onto the system to produce guided-spin flow in their least resistive directions, resulting in a spin-dependent current generation specifically in the asymmetric antiparallel magnetic state. Strength of the interfacial exchange interaction We start by analyzing the exchange interaction at the interface between a magnetic insulator and its neighbouring free electrons. The magnitude of the exchange splitting has been formulated previously [22] , [27] , [28] . We follow the same approach to evaluate the expected exchange splitting in our EuS/Al system. EuS is a well-studied SF material with a Curie temperature of 16.6 K. The effective Zeeman splitting of the Al conduction electrons can be expressed as: where c is the fractional interface ratio of the Eu 2+ ions relative to that of the Al conduction electrons, J is the exchange interaction energy, and S Eu =7/2 is the spin of Eu 2+ ions. Since we are dealing with ultrathin Al films at low temperatures, all the Al conduction electrons are expected to participate equally in the exchange interaction with the interface Eu 2+ ions. Therefore, c is simply the ratio of the sheet density of Eu 2+ ions to that of Al conduction electrons, ~ c =0.031/ t , where t is the nominal Al film thickness in nanometre. We assume bulk densities and three conduction electrons per Al atom in this estimation. From the above discussion, we see that the exchange splitting naturally has a 1/ t dependence on the nominal Al layer thickness [22] , [28] . Indeed, the spin splitting in Al owing to the exchange interaction at the EuS/Al interface has been shown to be inversely proportional to the Al layer thickness [25] , clearly indicating that the observed exchange values are owing to the interface effect averaged over all the sheet carriers per unit area. From the known value of Δ ~0.26 meV (~4.5 T internal field) for a 4 nm Al film [25] , we deduce the magnitude of the exchange constant J ~9.6 meV, consistent with the values determined from other methods [26] . We also know that the spin orientation of polarized conduction electrons is opposite to those of the rare-earth ions, which was well-documented in earlier NMR studies [29] , [30] . Therefore, the energy of a conduction electron will be exchange-shifted downwards when its spin aligns antiparallel with that of the rare-earth ion, and vice versa. When such exchange splitting is confined on a Coulomb island with negligible intrinsic spin relaxation, any non-equilibrium perturbations on the island will produce long-lived spin excitations, and spin relaxation can only occur through communication with external electrodes. We next show that we can use the spin sensitive tunnel barrier, that is, a spin filter, to directly probe the energy levels on these two-spin channels, which then allows us to harvest excitations from extrinsic sources to produce directional spin and charge flow. 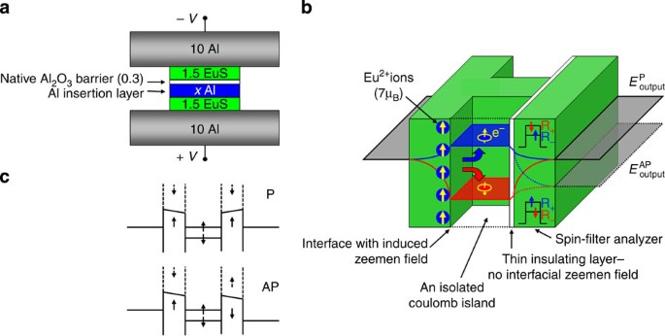Figure 1: Device layout and electronic energy profile. (a) Illustration of the device layout, with thickness in nanometre. The first (bottom) EuS layer makes a clean interface with the middle Al insertion layer, and the second (top) EuS layer is separated from the insertion layer by a thin native oxide to eliminate exchange coupling. (b) Electron energy diagram across the junction: the first (left) EuS layer creates the electron energy-splitting in the insertion layer, with the energy levels of spin-up electrons pushed upwards, while those of the spin-down electrons are pushed downwards; the second (right) EuS layer functions as the spin analyzer, and can be simplified as two resistors corresponding to the two respective spin channels. In practice, the inserted ultrathin layer forms clusters that can be treated as Coulomb islands (illustrated here as a channel separated from the neighbours with an energy barrier); a natural oxide ~2 monolayers (3 Å) forms on the Al surface before the second EuS layer is laid down, which functions to block the exchange field at this interface. The electron energy levels in the output electrode () are evaluated using Equation (2). (c) Simplified-energy diagram for an ideal condition (infinite minority barrier height, that is, perfect spin filtering) to illustrate the potential difference across the device. EuS/Al 2 O 3 /Al/EuS device structure Figure 1a illustrates the device structure consisting of two 10 nm thick Al electrodes on either side of the EuS/Al 2 O 3 /Al/EuS heterostructure. The heterostructure consists of two 1.5 nm thin EuS layers separated by a middle Al insertion layer that is covered by a 0.3 nm thin Al 2 O 3 native oxide. In practice, the ultrathin Al layer breaks up into isolated nanoclusters within the barrier (evidence of Coulomb confinement on the islands are shown in the Supplementary Fig. 1 and Supplementary Note 1 ), but on an average, the exchange splitting for the entire device can still be evaluated from Equation (1) because it is solely determined by the ratio between the total number of electrons and the number of Eu ions. One side of the Al island is in direct contact with EuS and experiences exchange coupling, while the thin natural Al 2 O 3 barrier eliminates exchange coupling between the Al and the EuS at the other interface. The conduction electrons in the Al thus experience an exchange interaction only at the clean contact side with the EuS, which generates an effective Zeeman splitting on the Al energy levels. The last electron on an island with odd occupancy can have two closely placed spin levels for its spin to shuffle back and forth under external excitations (illustrated in Supplementary Fig. 2 ), while the last electron on an island with even occupancy can hardly flip its spin owing to the large Coulomb charging energy required (explained in more details in Supplementary Note 2 ). Owing to the random physical and chemical environment around the Coulomb islands, they can experience different offset voltage on their energy levels. Here we first consider dots with their offset voltage close to zero because these are most susceptible to external excitations and contribute most to our experiment. On the other hand, our conclusions do not change in the presence of offset voltage distribution on the islands, as long as one spin channel is uniformly higher than the other one across all the islands (see Supplementary Fig. 3 and Supplementary Note 2 ). Figure 1: Device layout and electronic energy profile. ( a ) Illustration of the device layout, with thickness in nanometre. The first (bottom) EuS layer makes a clean interface with the middle Al insertion layer, and the second (top) EuS layer is separated from the insertion layer by a thin native oxide to eliminate exchange coupling. ( b ) Electron energy diagram across the junction: the first (left) EuS layer creates the electron energy-splitting in the insertion layer, with the energy levels of spin-up electrons pushed upwards, while those of the spin-down electrons are pushed downwards; the second (right) EuS layer functions as the spin analyzer, and can be simplified as two resistors corresponding to the two respective spin channels. In practice, the inserted ultrathin layer forms clusters that can be treated as Coulomb islands (illustrated here as a channel separated from the neighbours with an energy barrier); a natural oxide ~2 monolayers (3 Å) forms on the Al surface before the second EuS layer is laid down, which functions to block the exchange field at this interface. The electron energy levels in the output electrode ( ) are evaluated using Equation (2). ( c ) Simplified-energy diagram for an ideal condition (infinite minority barrier height, that is, perfect spin filtering) to illustrate the potential difference across the device. Full size image Figure 1b illustrates the electron energy levels in the device structure. Here electrons are injected into the left-hand (bottom) EuS barrier, pass through the Al, and are spin-filtered as they pass through the right-hand (top) EuS barrier. To analyze the electrical conduction of the device, we use the two-spin current model, treating the SF barriers as a set of spin-dependent resistors R + ( R − ) for the spin channels facing the higher (lower) energy barrier [31] , illustrated in the figure’s right-hand EuS barrier. When no net charge current flows across the structure in the equilibrium state, we have: Here and are the electron energy levels in the right-hand detector electrode in the spin parallel (P) and antiparallel (AP) configurations, respectively. After some algebra, we obtain the measured voltage shift between these two states as, where is simply the SF efficiency, that is, the percentage of the spin polarized conductance in the total conductance. We see that the experimentally measured voltage shift between the two spin states is just the interfacial exchange splitting modulated by the SF efficiency. Note that in our definition of voltage polarity ( Fig. 1a ), the higher electron energy level at the top (right-hand on Fig. 1b ) electrode corresponds to a higher measured voltage on the voltmeter. The physics behind this is easy to understand: since the SF barrier preferentially allows electrons with one spin-type to communicate across it, the detector electrode is therefore only probing the energy level of this spin-type. Reversing the magnetization orientation of the SF layer allows for the detection of the opposite spin-type. In the ideal situation, a perfect spin-filter would have an infinitely tall spin-minority barrier forbidding any electron communications on this channel, and the Fermi level across the device would look like the one illustrated in Fig. 1c . Specifically, on the AP configuration, the internal spin splitting can fully propagate into the electrodes. 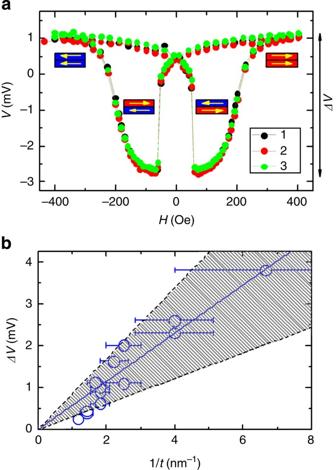Figure 2: Spin-dependent voltage measurement. (a) Measured spontaneous spin-dependent voltage corresponding to the majority and minority spin channels as a function of applied magnetic field. The measurements were performed in a simple two-terminal configuration, and results of three different junctions on the same chip are plotted together for comparison, whereT=1 K andx=0.15 nm. (b) Dependence of the measured spin-dependent voltage shift on the inverse Al insertion layer thickness atT=1 K. Shaded area illustrates the error associated with the slope determination. In practice, however, SF barriers are never perfect and the detected energy level is thus modified by the SF efficiency α. Spin-controlled spontaneous voltage Figure 2a shows data for the measured spontaneous voltage across several device junctions, while toggling the system with magnetic field H between spin-parallel and -antiparallel alignment. Two well-defined voltage states are clearly visible, corresponding to the up and down-spin channels, respectively. The measured voltage is higher in the parallel magnetic configuration, which confirms that the indirect exchange interaction indeed prefers to align electron spins antiparallel to those of the rare-earth ions. The largest voltage difference (Δ V ) measured was about 3.8 mV for the thinnest Al insertion layer that we were able to fabricate. To put things into perspective, this corresponds to an effective Zeeman field of over 60 T in strength operating only on the electrons’ spin degrees of freedom, not on their orbitals. However, for the nominal thickness of 0.15 nm Al, we would expect, from Equation (1), that the internal exchange splitting (2 Δ ) to be around 14 meV. The difference is thus a direct measure of the non-ideal SF efficiency α, as pointed out in Equation (3). By varying the inserted Al layer thickness, we see from Fig. 2b that the observed energy-splitting indeed follows a 1/ t dependence. Using the best fit to all the data, we find the SF efficiency to be about 28±13%. The large error bar is associated with the experimental uncertainty in determining the nominal Al thickness, given that the measured voltage is a highly sensitive function of this thickness. The seemingly small SF efficiency value can mostly be attributed to the thinness of EuS barrier that we used in this experiment (1.5 nm) compared with that reported in literature (80% through 2.5 nm EuS) [15] , because the SF efficiency depends strongly on the SF barrier thickness [32] . Moreover, from the shape of the V ( H ) curve in Fig. 2a it is clear that a complete antiparallel alignment is not yet achieved between the two SF layers (absence of a flat-bottomed minima). Considering that the maximum obtained tunnelling MR (TMR) in transport measurements is only 40% with 1.5 nm EuS [19] , a rough estimate using Julliere’s tunnelling model leads to a maximum detectable SF efficiency of 40% in the current devices. Figure 2: Spin-dependent voltage measurement. ( a ) Measured spontaneous spin-dependent voltage corresponding to the majority and minority spin channels as a function of applied magnetic field. The measurements were performed in a simple two-terminal configuration, and results of three different junctions on the same chip are plotted together for comparison, where T =1 K and x =0.15 nm. ( b ) Dependence of the measured spin-dependent voltage shift on the inverse Al insertion layer thickness at T =1 K. Shaded area illustrates the error associated with the slope determination. Full size image In the above analysis we have treated the exchange split levels on the Al cluster as two separate energies. If the Al insertion layer were electrically continuous, we would have a single Fermi level across the whole layer (see Supplementary Fig. 4 ), and the Zeeman field would only shift the spin-up and spin-down band bottom (like in a ferromagnet under exchange field). In that case the spin-up and -down electrons would populate up to the same energy level despite their population being somewhat different under the localized Zeeman field. This would have prevented us from observing the spin voltage signal across the device. Clustering of the ultrathin Al film into nano-islands completely changes the above picture. We can readily estimate the order of magnitude of charging energy on these Al islands. EuS has a relative dielectric constant 13.1 (ref. 33 ), so for a typical Al island size ~0.3 nm thick with a lateral size of 3 nm, the island capacitance is in the order of atto-farads, and the charging voltage is in the order of 10–100 mV (the aspect ratio of a typical island is based on AFM measurements of the grain size for 4 nm thick films, whereas the actual grain size is not critical as explained below). Therefore, we are dealing with electrons crossing an individual island one at a time. Each island has a quantized single electron level that is spin split owing to the exchange field from EuS, and the Fermi level roughly lies in the middle. It implies that there is a mixture of up-electron occupancy and down-electron occupancy across the islands, and they constantly shuffle between these two situations through communication with the electrodes. When that occurs, the up electrons, occupying higher energy levels, will tend to drag the detection electrode voltage downwards (as the electron charge is negative), while the down-electrons drag the voltage upwards. Also, through the same process, an up-spin electron on the island is exchanged with a down-spin electron, creating an effective spin-flipping process for the electrons on the island. Despite the expected island-to-island variations, up-spin electrons universally emerge at higher energies than down-spin electrons, by 2 Δ on an average. With the existence of two distinguishable spin energy levels, a SF barrier will selectively allow only one type of spin to communicate through (under ideal condition), and thereby enable selection of the desired spin channels. We want to emphasize that, although Coulomb blockade was used in our studies to provide discrete single electron energy levels, the phenomena we observed are not associated with Coulomb blockade itself. Any mechanism that can generate an isolated single electron energy level, coupled with a Zeeman splitting, would lead to the same results. We note that the precise size of the Coulomb islands does not matter here, as long as all other Coulomb levels are well separated from the electron level of interest, thus they are not accessible and will not contribute to the transport processes. Energy harvesting From the above discussions, we see that a spin-dependent voltage, albeit quite small, is spontaneously generated across a multilayer device. This makes it highly desirable to harvest the spin current using such a system. By connecting the two terminals of a device with a pico-ammeter and a load resistor in series, we can monitor the output current levels in the P and AP spin configurations. For a device with 0.6 nm Al insertion layer, the measured current difference (Δ I ) between the two magnetic states as a function of the load is shown in Fig. 3 . The maximum power consumption at the load is estimated to be about 27 fW. For devices with thinner Al insertion layers, the achievable power output is significantly diminished by the large internal impedance, as the device resistance goes up enormously and the output current approaches zero. 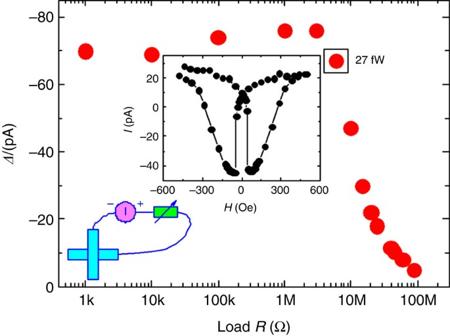Figure 3: Spin-dependent current measurement. Induced spin-dependent current in the presence of a resistance load. Inset shows the measurement setup and measuredI(H) curve with a 6 MΩ load resistor. Data were taken atT=1 K forx=0.15 nm. Figure 3: Spin-dependent current measurement. Induced spin-dependent current in the presence of a resistance load. Inset shows the measurement setup and measured I ( H ) curve with a 6 MΩ load resistor. Data were taken at T =1 K for x =0.15 nm. Full size image From the above experiments, we see that we can induce and detect a spin-dependent voltage across our device, and that the spins have a preferred direction of flow owing to the unique energy barrier profiles, which is accompanied with a finite amount of power output from the device. We can estimate the magnetostatic energy stored in our device. The electromotive force could potentially behave as a non-equilibrium energy source [34] , [35] . An applied field of strength ~200 Oe is needed to return the system from antiparallel back to parallel configuration, thus the total available magnetostatic energy is estimated to be 3.7 nJ cm −2 . This, however, can only support the energy output of our system for ~10 s. We thus attribute the energy harvested to extrinsic thermal and charge fluctuations, which are the sources for excitations and state shuffling. The device harvests fluctuations from the environment and converts them into useful energies. We further demonstrated that control devices that do not contain the Al insertion layer do not show any spontaneous voltage shift between the states, and samples with reversed sample growth order showed exactly reversed-voltage signals (see Supplementary Fig. 5 and Supplementary Note 3 ). It is worth pointing out here that reversing the layer order does not change junction impedance, or temperature gradient direction, if any. These verifications confirm that the observations are indeed originating from the samples, rather than related to experimental artifacts. In the AP state, we observed a spontaneous decay of the observed signal with a time scale on the order of 10 4 s. We attribute such a slow decay to the internal magnetic relaxation towards the more stable-P state, the true ground state of the system (see Supplementary Figs 6, 7 and Supplementary Note 4 ). Further evidence of the existence of the internal spin-level splitting can be seen from tunnelling measurements, where an externally applied voltage drives a current through the device. When at least some portion of the aligned spin population is conserved in the transport process, an MR is developed. Understandably, the inserted Al lowers the overall junction MR since the tunnelling electrons can spend an appreciable amount of time at the inserted layer and have more chance to be spin-scattered. 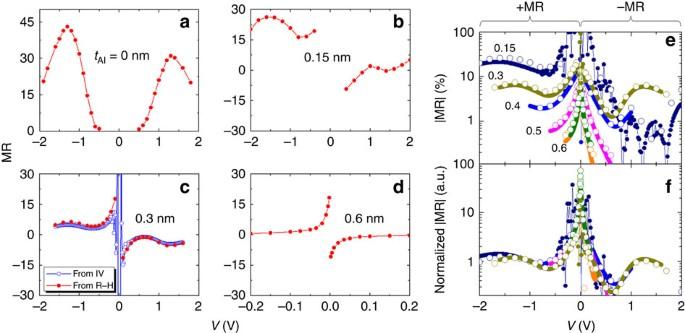Figure 4: MR across the device. MR bias dependence in the presence of spin-dependent voltage shift using standard four-terminal measurements with constant voltage atT=1 K. (a–d) MR in devices with nominallyx=0, 0.15, 0.3, 0.6 nm inserted Al. (e) MR bias dependence plotted together. Note thatabsolutevalues are plotted here on a logarithm scale. Open symbols indicate values determined from measured R(H) loops, while closed symbols were deduced from IV curves. (f) Replot of the same curves after normalization. Figure 4a shows the TMR of a standard double SF tunnel junction with a fully-oxidized Al 2 O 3 spacer layer (nominally 0.25 nm Al deposited; qualitatively the same results were obtained in ref. 19 ). The TMR shows the standard bias dependence expected in such junctions, and hence we conclude that the oxidation process fully consumed the deposited 0.25 nm Al. For samples with nominally more Al deposited, the TMR bias dependence begins to deviate from the above standard behaviour. Figure 4b–d show results from junctions that were deposited in the same deposition run but with progressively thicker Al insertion layers. Two unique features develop in their bias dependence: (i) inverse MR was observed under positive bias, and (ii) the MR diverges around zero bias. In Fig. 4e , the magnitude of MR is plotted on a logarithm scale with respect to bias voltage, and, after normalization, they collapse onto a universal curve ( Fig. 4f ). This suggests that the observed MR bias dependence has the same underlying physical mechanism—a spin-dependent voltage shift. Further discussion of this universal curve are included in Supplementary Fig. 8 and Supplementary Note 5 . Finally, we note that the robustness of the TMR reversal up to high voltages clearly rules out possibilities of small measurement artifacts from the experimental setup. Figure 4: MR across the device. MR bias dependence in the presence of spin-dependent voltage shift using standard four-terminal measurements with constant voltage at T =1 K. ( a – d ) MR in devices with nominally x =0, 0.15, 0.3, 0.6 nm inserted Al. ( e ) MR bias dependence plotted together. Note that absolute values are plotted here on a logarithm scale. Open symbols indicate values determined from measured R(H) loops, while closed symbols were deduced from IV curves. ( f ) Replot of the same curves after normalization. Full size image In summary, we used the SF effect to directly probe the exchange-induced spin splitting present at the magnetic insulator/metal interface. This allowed us to quantify both the exchange-splitting amplitude and the effectiveness of SF—two important intrinsic properties of magnetic insulators. We further demonstrated that by controlling the spin-dependent energy profiles, spin and charge flow can be controlled, enabling the useful control of spin information in electronic devices and the possibility of harvesting work from the system. Sample layout The basic structure we investigated (see Fig. 1 ) consists of a thin film stack on glass substrate (thickness in nm): 10 Al/1.5 EuS/ x Al/0.3 Al 2 O 3 /1.5 EuS/10 Al. The thickness x of the metallic Al insertion layer sandwiched between the two EuS SF layers is varied from 0.1–0.8 nm. Materials deposition Al was deposited by thermal evaporation, whereas EuS was deposited by e-beam evaporation. To have different coercivities for the two EuS layers, the first layer was deposited at liquid nitrogen temperature, whereas the second one was deposited at room temperature. The Al insertion layer makes direct contact with EuS at its bottom interface, while it is isolated from the top EuS by an intentionally-formed Al 2 O 3 natural barrier during the warm up process (1.5 h). Such configuration allows for exchange interactions between Eu 2+ ions and conduction electrons in Al [11] , [22] , [23] to occur at the bottom interface but not at the top interface. The oxidation process consumes about 0.25 nm of Al metal to form 0.3 nm (two monolayers) of Al 2 O 3 : the thickness 0.3 nm was deduced since below this thickness we no longer observe any signatures of metallic clusters in our devices, indicating Al was fully consumed into Al 2 O 3 . In this study, the nominal Al insertion layer thickness x is the actual deposited thickness minus 0.25 nm. Device measurement The active junction area was 200 × 200 μm 2 . Our measurement setup is based on voltage sensing, and the current is determined by the voltage drop across a series resistor. The junction impedance of the devices, which depends on the Al insertion layer thickness and bias voltage, ranged from tens of kΩ to tens of MΩ. Our magnetic field sweep rate was constant,~5 Oe s −1 , rendering the typical measurement time of 5 min per loop. The impedance of the nanovoltmeter is specified at 10 GΩ, and the measurement was performed with junction leads connected through pressed In contact and Cu wiring. The devices were fully submerged in a superfluid helium bath. Open circuit voltage was measured with two terminals of the junction device connected to the voltmeter inputs. Current flowing through the device was obtained by measuring the voltage drop across the resistor inserted in series with the device. Ferrite radio frequency filters are attached to the measurement cables to eliminate the pickup of undesired radio frequency energies from the environment, however, internal fluctuations from the instruments were not shielded. TMR measurements were done by a four-terminal method, passing a current through two contacts across the device and recording its voltage response on two other contacts. All these different configurations yielded self-consistent results, eliminating possibilities of measurement artifacts. How to cite this article: Miao, G.-X. et al. Spin regulation in composite spin-filter barrier devices. Nat. Commun. 5:3682 doi: 10.1038/ncomms4682 (2014).